Toward atomically-precise synthesis of supported bimetallic nanoparticles using atomic layer deposition Multi-metallic nanoparticles constitute a new class of materials offering the opportunity to tune the properties via the composition, atomic ordering and size. In particular, supported bimetallic nanoparticles have generated intense interest in catalysis and electrocatalysis. However, traditional synthesis methods often lack precise control, yielding a mixture of monometallic and bimetallic particles with various compositions. Here we report a general strategy for synthesizing supported bimetallic nanoparticles by atomic layer deposition, where monometallic nanoparticle formation is avoided by selectively growing the secondary metal on the primary metal nanoparticle but not on the support; meanwhile, the size, composition and structure of the bimetallic nanoparticles are precisely controlled by tailoring the precursor pulse sequence. Such exquisite control is clearly demonstrated through in situ Fourier transform infrared spectroscopy of CO chemisorption by mapping the gradual atomic-scale evolution in the surface composition, and further confirmed using aberration-corrected scanning transmission electron microscopy. Bimetallic nanoparticles often show unique electrical, magnetic, optical and catalytic properties that are distinct from those of their parent metals, making them a new class of materials with enhanced properties because of synergistic effects [1] , [2] , [3] , [4] , [5] , [6] , [7] . These materials have gained broad interest for a range of applications. In particular, bimetallic nanoparticles supported on oxides (or carbon) have been used extensively in catalytic [2] , [4] , [7] , [8] , [9] , [10] , [11] , [12] and electrocatalytic [5] , [13] , [14] , [15] , [16] applications such as hydrocarbon reforming, water-gas-shift and fuel cells. Traditional methods for bimetallic nanoparticle synthesis such as successive impregnation or co-impregnation often fail to provide precise control over composition and structure, yielding a mixture of monometallic and bimetallic particles with various compositions [2] , [7] , [17] . This heterogeneity will obfuscate any effort to link properties to structural or compositional changes, and can significantly reduce the catalytic performance. Monnier et al. [18] recently utilized electroless deposition to promote the selective growth of a second metal on the surface of a pre-existing metal without forming isolated clusters of the second metal on the catalyst support. However, the coverage of the second metal was limited to the submonolayer region, and the synthesis of well-mixed alloys using this approach might be challenging. Consequently, a more general method for bimetallic nanoparticle synthesis with atomically precise control is still missing. Atomic layer deposition (ALD) is a variation of chemical vapour deposition, wherein thin films are grown via a sequence (usually binary) of self-limiting chemical reactions between precursor vapours and the surface [19] , [20] , [21] . The self-limiting character of the reactions makes it possible to achieve uniform deposits on high surface area or porous solids [22] , [23] , [24] . Hence, the design and synthesis of advanced nanoscale catalysts become possible through independent control over the structure and composition of the underlying support, the catalytically active sites and the protective overlayer [25] , [26] , [27] . ALD has proven successful for the controlled synthesis of supported monometallic catalysts [24] , [26] , [28] . Although there have been a few reports of bimetallic nanoparticles by ALD, these have been limited to the case where the two metals share a similar surface chemistry and deposition temperature [29] , [30] , and no strategy was provided for controlling the deposition of the secondary metal selectively on the primary metal nanoparticle but not on the support to exclude monometallic formation. Very recently, Kessels et al. [31] , reported the selective ALD of a Pt shell on Pd particles supported on planar substrates using a low oxygen pressure at 300 °C, where the Pd core was prepared at 100 °C using a H 2 plasma as the reducing agent. In addition, they reported the selective ALD of a Pd shell on Pt nanoparticles using H 2 as the reductant at 100 °C, where the Pt core was prepared using a high oxygen pressure at 300 °C. However, the use of a plasma renders the method unsuitable for high surface area or high aspect ratio substrates where the radical species in the plasma would recombine before reaching the inner surfaces. Moreover, the need to perform the growth of the two metals at different temperatures is inconvenient, and makes the growth of bimetallic alloy nanoparticles, where the two ALD metal processes must be frequently alternated, practically impossible. Here we report a general strategy for synthesizing supported bimetallic nanoparticles by ALD that overcomes these limitations. By properly selecting the deposition temperature and the appropriate co-reactant, we achieve selective deposition of the second metal only on the surfaces of the first metal without the need for a plasma, which is illustrated using in situ quartz crystal microbalance (QCM) measurements. Moreover, by maintaining a constant temperature for the multiple metal ALD processes, the synthesis of well-mixed alloy nanoparticles is accomplished. In situ Fourier transform infrared spectroscopy (FTIR) of CO chemisorption clearly demonstrates the atomically precise control offered by ALD through mapping the atomic-scale evolution of the nanoparticle surface composition after every ALD cycle of the selectively deposited secondary metal, and from these measurements both the nanoparticle structure and the stability are inferred at elevated temperatures. Moreover, aberration-corrected scanning transmission electron microscopy (STEM), along with elemental line profile analysis, confirms the composition and structure of the bimetallic nanoparticles. Our results demonstrate a general methodology for the atomically precise, low temperature synthesis of supported bimetallic or multi-metallic nanoparticles on both planar and porous surfaces suitable for catalysis and other applications. Low temperature selective metal ALD We first employed in situ QCM measurements to establish the appropriate conditions to accomplish the selective deposition of ALD metals on metal surfaces while avoiding growth on oxide surfaces. In these studies, a primary metal or oxide starting surface was first deposited onto the quartz crystal sensor by ALD, and then the initial growth behaviour of the secondary metal was recorded. A variety of deposition temperatures, co-reactants and pulse-sequencing strategies were explored to achieve the desired selectivity. 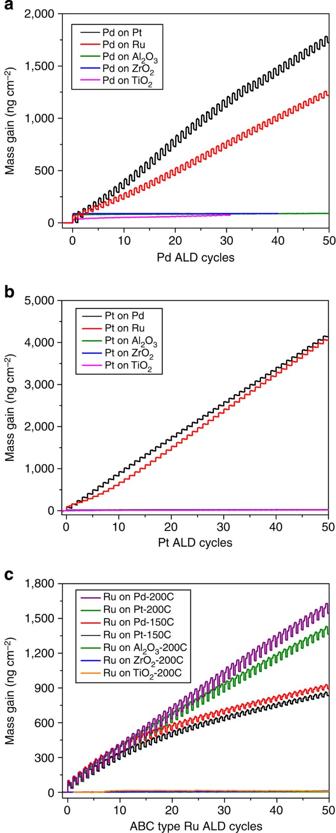Figure 1:In situQCM measurements of ALD on metal and oxide surfaces. (a) Pd ALD on Pt, Ru, Al2O3, TiO2and ZrO2using Pd(hfac)2and H2at 150 °C. (b) Pt ALD on Pd, Ru, Al2O3, TiO2and ZrO2using MeCpPtMe3and O2at 150 °C. (c) ABC-type Ru ALD on Pd and Pt at 150 and 200 °C, and on Al2O3, TiO2and ZrO2at 200 °C using Ru(EtCp)2, O2and H2. Figure 1 summarizes the successful processes we discovered. On Pt or Ru metal surfaces, Pd ALD using Pd(II) hexafluoroacetylacetonate (Pd(hfac) 2 ) and H 2 at 150 °C exhibits linear growth without any nucleation delay ( Fig. 1a ). A slightly higher initial growth rate was obtained on Pt than on Ru. In contrast, no Pd growth was observed under these conditions on Al 2 O 3 , TiO 2 or ZrO 2 surfaces except for the small mass uptake during the first Pd(hfac) 2 exposure (also seen in Supplementary Fig. 1 ). Similarly, Pt ALD showed linear growth on Pd and nearly on Ru surfaces using trimethyl(methylcyclopentadienyl)-platinum(IV) (MeCpPtMe 3 ) and O 2 at 150 °C ( Fig. 1b ). The Pt ALD was slightly inhibited initially on the Ru surface. Again, negligible Pt growth was observed on the Al 2 O 3 , TiO 2 and ZrO 2 surfaces under the same conditions (also seen in Supplementary Figs 2 and 3 ) [32] . Figure 1: In situ QCM measurements of ALD on metal and oxide surfaces. ( a ) Pd ALD on Pt, Ru, Al 2 O 3 , TiO 2 and ZrO 2 using Pd(hfac) 2 and H 2 at 150 °C. ( b ) Pt ALD on Pd, Ru, Al 2 O 3 , TiO 2 and ZrO 2 using MeCpPtMe 3 and O 2 at 150 °C. ( c ) ABC-type Ru ALD on Pd and Pt at 150 and 200 °C, and on Al 2 O 3 , TiO 2 and ZrO 2 at 200 °C using Ru(EtCp) 2 , O 2 and H 2 . Full size image Ru ALD has been accomplished previously using bis(ethylcyclopentadienyl)ruthenium (Ru(EtCp) 2 ) and O 2 at 300 °C (ref. 33 ), here we found that Ru ALD does not proceed below 200 °C ( Supplementary Fig. 4a ). To achieve Ru ALD at 150 °C where the Pt and Pd ALD were selective, we adopted an ABC-type strategy using the exposure sequence: Ru(EtCp) 2 , O 2 and H 2 . In this process, the Ru(EtCp) 2 should undergo dissociative chemisorption on the existing Ru surface, the O 2 is expected to burn off the EtCp ligand forming Ru oxide, and the H 2 should reduce the Ru oxide to Ru metal. In agreement with this expected mechanism, the ABC sequence yielded Ru ALD at much lower temperatures and provided ~0.21 Å per cycle (22.4 ng cm −2 per cycle) at 200 °C and 0.1 Å per cycle (10.5 ng cm −2 per cycle) at 150 °C ( Supplementary Fig. 4b ). Moreover, the ABC Ru ALD enabled selective growth on Pd or Pt surfaces but not on Al 2 O 3 , TiO 2 and ZrO 2 surfaces at 200 °C ( Fig. 1c ). The higher initial Ru growth rates observed on the Pd and Pt surfaces at 150 °C suggest that these metals facilitate the Ru nucleation and growth. Figure 1 demonstrates the selective ALD of secondary metals on primary metal surfaces, but of course a compatible ALD process is also required to deposit the primary metal on the oxide support to initiate the bimetallic growth. Fortunately, Pd ALD can be accomplished on oxide surfaces at 150 °C using HCHO as the coreactant ( Supplementary Fig. 1 ) [28] , [34] . Similarly, Pt ALD can be achieved on oxide surfaces at the low temperatures needed for selective growth of the secondary metal using O 3 as the coreactant ( Supplementary Fig. 3 ). This strategy, when coupled with the saturating reactions of the secondary metal on the primary metal surface leads exclusively to bimetal nanoparticles without forming monometallic nanoparticles of the primary or the secondary metal. Using the methods described above, bimetallic core-shell nanoparticles can in principle be formed on oxide surfaces with precise control over the shell thickness by adjusting the number of ALD cycles for the secondary metal. The ALD of well-mixed bimetallic alloy nanoparticles could also be accomplished by alternating between the ALD processes for the individual metals, but certain requirements must be satisfied. Besides the requirement of the selective deposition of each metal component, the surface chemistries for the two components must be mutually compatible and ALD of two metals should proceed at the same temperature for practicality. 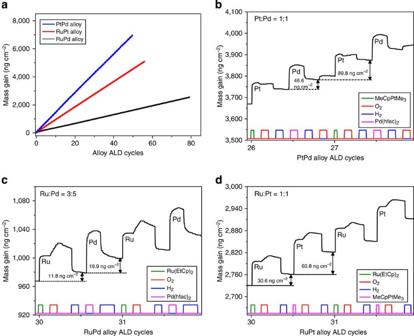Figure 2:In situQCM studies of low temperature metal alloy ALD. (a) Linear growth of PtPd, RuPd and RuPt alloys by alternating between the ALD processes for the two metals. (b) Detailed mass changes during two PtPd alloy supercycles. (c) Detailed mass changes during two RuPd alloy supercycles. (d) Detailed mass changes during two RuPt alloy supercycles. The sequential exposure steps of each reactant are shown as columns in color at the bottom of each figure, nitrogen purge step is in between the columns. Figure 2 shows in situ QCM measurements of well-mixed metal alloy ALD for all possible combinations: PdPt, RuPd and RuPt. The PdPt, RuPd and RuPt alloy ALD yield linear growth at 150 °C as shown in Fig. 2a . The PdPt well-mixed alloy was accomplished using the sequence: MeCpPtMe 3 -O 2 -H 2 -Pd(hfac) 2 -H 2 -O 2 (ABC-type Pt with ABC-type Pd ALD). The H 2 exposure after the O 2 exposure in each Pt ALD cycle reduces the surface and enhances the Pd growth. In the absence of the extra H 2 exposure, the Pd ALD is suppressed ( Supplementary Fig. 5 ). This is probably due to Pd(hfac) 2 dissociation by the chemisorbed oxygen. Similarly, an O 2 exposure added after the H 2 exposure in each Pd ALD cycle oxidizes the surface to facilitate the subsequent MeCpPtMe 3 adsorption for the Pt ALD. 1c-Pt ALD followed by 1c-Pd ALD yielded a Pd:Pt mole ratio of about 1:1 ( Fig. 2b ). Combining ABC-type Pt with AB-type Pd ALD barely changed the overall growth rate for the alloy, but changed the mole ratio to Pd:Pt=4:3 ( Supplementary Fig. 6 ). Well-mixed RuPd alloy growth was achieved using the ALD sequence: Ru(EtCp) 2 -O 2 -H 2 -Pd(hfac) 2 -H 2 at 150 °C, which gave a Ru:Pd mole ratio of about 3:5 ( Fig. 2c ). Similarly, a well-mixed RuPt alloy was accomplished using the sequence: Ru(EtCp) 2 -O 2 -H 2 -MeCpPtMe 3 -O 2 -H 2 at 150 °C, which yielded a Ru:Pt mole ratio of 1:1 ( Fig. 2d ). It is notable that the ABC-type Ru ALD showed a higher growth per cycle during the RuPt alloy ALD (30.6 ng cm −2 , Fig. 2d ), than on itself (10.5 ng cm −2 , Supplementary Fig. 4 ). Similar behaviour is also seen in Fig. 1c , where the Ru growth per cycle is higher initially on the Pt surface, but then declines to a lower value following ~15 cycles where the surface has converted to Ru. Figure 2: In situ QCM studies of low temperature metal alloy ALD. ( a ) Linear growth of PtPd, RuPd and RuPt alloys by alternating between the ALD processes for the two metals. ( b ) Detailed mass changes during two PtPd alloy supercycles. ( c ) Detailed mass changes during two RuPd alloy supercycles. ( d ) Detailed mass changes during two RuPt alloy supercycles. The sequential exposure steps of each reactant are shown as columns in color at the bottom of each figure, nitrogen purge step is in between the columns. Full size image In situ CO chemisorption FTIR during ALD synthesis The QCM results in Figs 1 and 2 demonstrate that the atomically precise synthesis of supported bimetallic nanoparticles should be possible, wherein the composition, structure and size of the nanoparticles can be controlled by adjusting the ALD pulse sequence [27] . To validate this approach, we employed FTIR to interrogate the surface of the bimetallic nanoparticles after each ALD cycle of the secondary metal. FTIR of CO chemisorption has been widely used to characterize the surface composition of bimetallic nanoparticles [4] , [35] , [36] , [37] , [38] . By performing in situ FTIR measurements of CO chemisorption after each ALD cycle during the bimetallic nanoparticle synthesis, we can map the atomic-scale evolution of the surface composition and thereby infer the nanoparticle structure (for example, core-shell versus well-mixed alloy). 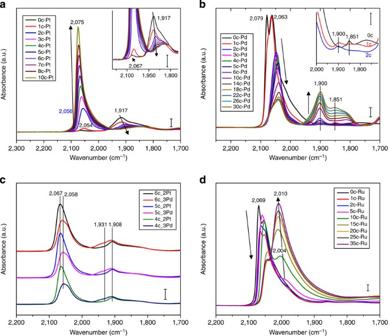Figure 3:In situCO chemisorption FTIR measurements during ALD process. (a) ALD of Pt shell on an ALD Pd/Al2O3sample at 150 °C. Scale bar, 1%, scale bar for the inset, 0.5%. (b) ALD of Pd shell on an ALD Pt/Al2O3sample at 150 °C. Scale bar, 3%, scale bar for the inset, 1%. (c) PtPd alloy ALD on an ALD Pt/Al2O3sample at 150 °C. Scale bar, 10%. (d) ALD of Ru shell on an ALD Pt/Al2O3sample at 200 °C. Scale bar, 2%. Figure 3a illustrates the growth of a Pt shell on an ALD Pd/Al 2 O 3 sample ( Supplementary Fig. 7 ), which was prepared using four ALD Pd cycles at 200 °C. The FTIR spectrum for CO adsorbed on the bare Pd/Al 2 O 3 sample ( Fig. 3a , 0c-Pt) showed a weak peak at 2,067 cm −1 and a strong peak at 1,917 cm −1 with a broad shoulder at around 1,850 cm −1 , which we assign to linear CO on steps/corners of the Pd nanoparticles and bridge/threefold-hollow CO on the Pd(111) facets, respectively [25] , [39] . After one Pt ALD cycle, the IR spectrum (1c-Pt) revealed that the linear CO intensity increased remarkably along with a red shift to 2,054 cm −1 , attributable to linear CO on Pt [40] ; meanwhile, the dominant peak at 1,917 cm −1 decreased and shifted to 1,913 cm −1 indicating a reduction in the concentration of surface Pd. With increasing Pt ALD cycles this trend continued: the intensity of the linear CO feature increased substantially but shifted to the blue while the bridging CO feature decreased in intensity and shifted to the red. After ~10 Pt ALD cycles, the bridge-bonded CO peak at 1,917 cm −1 on Pd disappeared, leaving only a weaker peak at 1,851 cm −1 , assigned to bridge-bonded CO on Pt [40] . This signals the completion of a continuous Pt shell on the Pd nanoparticle core. From Fig. 1b , the Pt mass added after 10 Pt ALD cycles corresponds to ~1.5 atomic monolayers (ML). Figure 3: In situ CO chemisorption FTIR measurements during ALD process. ( a ) ALD of Pt shell on an ALD Pd/Al 2 O 3 sample at 150 °C. Scale bar, 1%, scale bar for the inset, 0.5%. ( b ) ALD of Pd shell on an ALD Pt/Al 2 O 3 sample at 150 °C. Scale bar, 3%, scale bar for the inset, 1%. ( c ) PtPd alloy ALD on an ALD Pt/Al 2 O 3 sample at 150 °C. Scale bar, 10%. ( d ) ALD of Ru shell on an ALD Pt/Al 2 O 3 sample at 200 °C. Scale bar, 2%. Full size image Figure 3b shows the complementary in situ CO chemisorption FTIR studies for Pd ALD (Pd(hfac) 2 and H 2 ) on a Pt/Al 2 O 3 sample prepared using 1c Pt ALD at 300 °C. Before the Pd ALD, two dominant linear CO peaks at 2,079 and 2,063 cm −1 along with a broad shoulder at ~2,010 cm −1 were observed, which we assign to linear CO adsorbed on larger and smaller Pt nanoparticles, and low coordinated Pt atoms, respectively [40] ; a very weak bridge-bonded CO peak at ~1,851 cm −1 was seen, consistent with the literature. After one Pd ALD cycle, the IR spectrum (1c-Pd) revealed that the broad shoulder at 2,010 cm −1 disappeared, suggesting that Pd preferentially nucleated at the low coordination Pt surface sites. This finding is in excellent agreement with a recent theoretical study by Fortunelli et al. [41] in which Pd mainly decorated the steps and corners of the Pt shell in multi-shell PdPt alloy nanoparticles. Meanwhile, a new peak appeared at 1,900 cm −1 , which we assign to bridge-bonded CO on the PdPt mixture [37] . With increasing Pd ALD cycles, the linear CO on Pt continuously decreased in intensity and shifted to lower wavenumbers, implying that the number of surface Pt atoms diminished. Surprisingly, the 1,900 cm −1 peak remained and the characteristic bridge CO peak at 1,931 cm −1 for pure Pd surfaces was not observed even after 30 Pd cycles (~3.5 ML Pd). This finding suggests that Pt atoms diffuse to the surface during Pd ALD on the Pt core, to produce a Pd-rich PdPt shell. Next, the PdPt well-mixed alloy ALD was investigated through in situ CO chemisorption FTIR at 150 °C ( Fig. 3c ). First, a high density of Pt nanoparticles with less than 1 nm size were prepared on an alumina support using 12 Pt ALD cycles (MeCpPtMe 3 and O 3 , Supplementary Fig. 8 ). Next, ‘supercycles’ of the PdPt alloy ALD were performed comprising 3c-Pd ALD followed by 2c-Pt ALD, and CO chemisorption was performed after each 3c-Pd and 2c-Pt step to probe the surface composition. Figure 3c illustrates CO chemisorption spectra following the 4th, 5th and 6th supercycles. Following each of the 3c-Pd step, the linear CO peak on Pt is suppressed while the 1,931 cm −1 peak (bridge CO on Pd) increases, clearly demonstrating that Pd has covered a fraction of the surface Pt atoms. Similarly, each execution of the 2c-Pt step reversed these trends, indicating that Pt has covered some of the surface Pd atoms. These reversible changes in the spectral features persisted over multiple supercycles ( Fig. 3c and Supplementary Fig. 9 ), providing solid evidence for the formation of a well-mixed PdPt alloy. Figure 3d illustrates in situ CO chemisorption FTIR studies of Ru ALD on a Pt/Al 2 O 3 sample at 200 °C. A gradual increase in the Ru surface coverage was observed with increasing Ru ALD cycles as evidenced by the decease of linear CO on Pt and the appearance of a new peak at 2,010 cm −1 , which we assign to linear CO on Ru [38] . Similar to the observations in Fig.3b , Pt CO features persisted even after 35 Ru ALD cycles (~3 Ru ML), suggesting diffusion of Pt to the surface during the Ru ALD. Structures of the ALD bimetallic nanoparticles To further investigate the structures of the bimetallic nanoparticles, we utilized high-angle annular dark field (HAADF) aberration-corrected STEM. 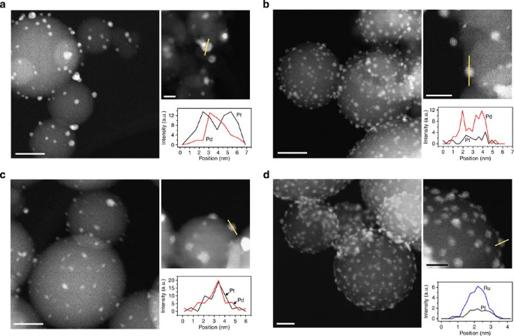Figure 4: Structures of ALD bimetallic nanoparticles. Representative aberration-corrected HAADF-STEM images and corresponding EDS line profiles of (a) 5Pd-core 15Pt-shell, (b) 12Pt-core 20Pd-rich-shell, (c) 12Pt10Pd alloy and (d) 1Pt-core 35Ru-rich-shell bimetallic nanoparticles on spherical alumina support. Figure 4a shows the Pd-core Pt-shell nanoparticles prepared on spherical alumina using 5c Pd ALD (Pd(hfac) 2 +HCHO) followed by 15c Pt ALD (MeCpPtMe 3 +O 2 ) at 150 °C that we designate: 5Pd-core 15Pt-shell (also seen in Supplementary Fig. 10 ). The 5Pd-core 15cPt-shell nanoparticles were mono-dispersed with a particle size of 2.7±0.63 nm. The STEM image with a higher magnification clearly demonstrated a Pd-core Pt-shell structure, where darker contrast is due to the atomically-lighter Pd and brighter contrast is attributed to the heavier Pt. The core-shell structure is further confirmed by the line profile analysis using STEM energy-dispersive spectroscopy (EDS). This observation is consistent with the in situ CO chemisorption FTIR studies. Figure 4: Structures of ALD bimetallic nanoparticles. Representative aberration-corrected HAADF-STEM images and corresponding EDS line profiles of ( a ) 5Pd-core 15Pt-shell, ( b ) 12Pt-core 20Pd-rich-shell, ( c ) 12Pt10Pd alloy and ( d ) 1Pt-core 35Ru-rich-shell bimetallic nanoparticles on spherical alumina support. Full size image Similarly, a sample of Pt-core Pd-shell bimetallic nanoparticles was prepared on spherical alumina using 12c Pt ALD (MeCpPtMe 3 +O 3 ) followed by 20c Pd ALD (Pd(hfac) 2 +H 2 ) at 150 °C (12Pt-core 20Pd-rich-shell). Well-dispersed PtPd bimetallic nanoparticles were formed with a particle size of 2.5±0.51 nm ( Fig. 4b and Supplementary Fig. 11 ). High-resolution STEM imaging along with EDS line profile analysis suggests a Pd-rich PdPt shell-Pt core structure, in agreement with the weak Pt features observed during the in situ CO chemisorption FTIR measurements even after 30c Pd ALD. Next, a well-mixed PtPd alloy sample was prepared on spherical alumina using 2c Pt ALD (MeCpPtMe 3 +O 3 ) at 150 °C to form subnanometer Pt nanoparticles as nucleation seeds, followed by ten PtPd alloy supercycles each comprised of 1c ABC Pd ALD (Pd(hfac) 2 +H 2 +O 2 ) and 1c ABC Pt ALD (MeCpPtMe 3 +O 2 +H 2 ). This sample is denoted as 12Pt10Pd alloy. In Fig. 4c , the STEM image shows well-dispersed nanoparticles with a size of 2.5±0.43 nm, and high resolution HAADF-STEM showed uniform contrast within each particle, indicating even mixing of Pt and Pd (also seen in Supplementary Fig. 12 ). Elemental line profile analysis provides further confirmation for the well-mixed PtPd alloy structure. Again, these findings corroborate the FTIR observations and illustrate the utility of the in situ FTIR technique for elucidating the bimetallic nanoparticle structure. The same Pt-core Ru-shell sample grown during the in situ FTIR CO chemisorption studies ( Fig. 3d ) was examined by STEM. As shown in Fig. 4d and Supplementary Fig. 13 , well-dispersed PtRu bimetallic nanoparticles were formed with a particle size of 1.9±0.37 nm, and the EDS line profile confirmed the presence of Pt atoms on the surface observed during the in situ CO chemisorption FTIR measurements. Thermal stability of the ALD bimetallic nanoparticles For practical purposes, it is important that the structure of the bimetallic nanoparticles should remain intact under catalytically relevant conditions. Here we briefly investigated the thermal stability of the bimetallic nanoparticles using in situ FTIR of CO chemisorption ( Fig. 5 ). We found that the well-mixed 12Pt10Pd alloy nanoparticles were stable at temperatures below 300 °C in N 2 , 10% O 2 or 10% H 2 indicated by the minor changes to the CO chemisorption features. While the linear CO on Pt surface (at 2,065 cm −1 ) decreased along with a considerable increase of the bridge CO on Pd (1,931 cm −1 ) after flowing 10% H 2 at 400 °C for 1 h ( Fig. 5a ), suggesting the migration of Pd atoms onto the alloy surface. Similarly, the 1Pt-core 35Ru-rich-shell nanoparticles were also found to be rather stable below 300 °C in both 10% O 2 and 10% H 2 . While above this temperature, Pt atoms started migrating to the particle surface, especially in flowing 10% H 2 , indicated by the considerable growth of linear CO on Pt at 2,048 cm −1 . 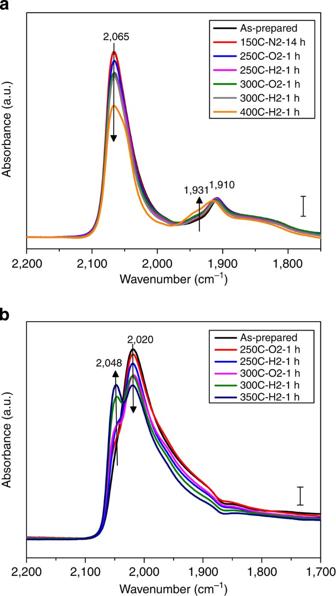Figure 5:In situCO chemisorption FTIR studies of particle stability. (a) The well-mixed 12Pt10Pd alloy nanoparticles treated at 150 °C in nitrogen for 14 h (150C-N2-14 h), then at 250, 300 and 400 °C in either 10% O2or 10% H2for 1 h (xC-O2-1h orxC-H2-1 h). Scale bar 5%. (b) 1Pt-core 35Ru-rich-shell nanoparticles treated at 250, 300 and 350 °C in either 10% O2or 10% H2for 1 h (xC-O2-1 h orxC-H2-1 h). Scale bar 3%. Figure 5: In situ CO chemisorption FTIR studies of particle stability. ( a ) The well-mixed 12Pt10Pd alloy nanoparticles treated at 150 °C in nitrogen for 14 h (150C-N2-14 h), then at 250, 300 and 400 °C in either 10% O 2 or 10% H 2 for 1 h ( x C-O2-1h or x C-H2-1 h). Scale bar 5%. ( b ) 1Pt-core 35Ru-rich-shell nanoparticles treated at 250, 300 and 350 °C in either 10% O 2 or 10% H 2 for 1 h ( x C-O2-1 h or x C-H2-1 h). Scale bar 3%. Full size image Challenges of supported bimetallic nanoparticle synthesis by ALD are that the deposition temperature and surface chemistry for the two metals are often different, and this complicates the task of combining them [27] . More importantly, no general strategy has emerged for achieving the selective growth of the secondary metal only on the primary metal surface while avoiding growth on the support to exclude monometallic nanoparticle formation. Using in situ QCM measurements, we demonstrated that selective deposition can be achieved by judiciously selecting the co-reactant and deposition temperature. For example, choosing H 2 instead of HCHO as the co-reactant for Pd ALD effectively suppresses Pd growth on oxide supports, while maintaining Pd growth on metal surfaces at 150 °C ( Supplementary Fig. 1 ). This selectivity might be further improved by treating the oxide surface with an alkyl alcohol before the Pd(hfac) 2 exposure to deactivate the oxide surface hydroxyl groups [34] , [42] . Reducing the deposition temperature is extremely effective at promoting selective ALD of the secondary metal. For instance, Pt ALD on TiO 2 , Al 2 O 3 , and ZrO 2 surfaces can be greatly suppressed by lowering the temperature from 300 to 150 °C ( Supplementary Figs 2 and 3 ). In contrast, Pt ALD at 150 °C on Pd and Ru surfaces is essentially identical to the growth at 300 °C ( Fig. 1b ). These contrasting behaviours for metal ALD on oxide versus metal surfaces facilitate the selective deposition at lower temperatures. In addition to the selectivity requirement discussed above that applies to the ALD of all bimetallic nanoparticles, the synthesis of well-mixed alloy nanoparticles mandates that the surface chemistries for the two components should be mutually compatible [29] , [43] . For instance, Pd ALD is a hydrogenation reaction process where surface H* are the active sites [44] , [45] ; while Pt ALD is a combustion reaction process, where surface O* are the active sites [46] , [47] . The direct combination of AB type Pd ALD (Pd(hfac) 2 +H 2 ) with AB type Pt ALD (MeCpPtMe 2 +O 2 ) causes decomposition of the hfac ligands on the O-terminated surface, which can produce carbon and fluorine contamination and also suppress the Pd growth ( Supplementary Fig. 5 ). In contrast, an O 2 exposure added after the H 2 exposure in each Pd ALD cycle can oxidize and O-terminate the surface in preparation for the subsequent MeCpPtMe 3 adsorption in the next Pt cycle. Similarly, a H 2 exposure added after the O 2 exposure in each Pt ALD cycle can reduce and H-terminate the surface for the subsequent Pd(hfac) 2 adsorption in the next Pd ALD cycle. Implementing this ABC strategy can satisfy the surface chemistries of each ALD process and facilitate the growth of the two components ( Supplementary Fig. 5 ). The higher growth rate observed for the alloy using this ABC method is beneficial for preparing supported PdPt alloy nanoparticles, because it further enhances the selective growth on the metal particle surface compared with the oxide support. We expect similar benefits from utilizing a Ru(EtCp) 2 -O 2 -H 2 -Pd(hfac) 2 -H 2 sequence for RuPd alloy ALD and a Ru(EtCp) 2 -O 2 -H 2 -MeCpPtMe 3 -O 2 -H 2 sequence for RuPt ALD. The selective growth of ALD metals on metal surfaces compared with oxide surfaces, coupled with the unique, self-limiting character of ALD allows atomically precise synthesis of supported bimetallic nanoparticles, a long-standing goal in catalyst synthesis. By tailoring the ALD pulse sequence, we can independently control the nanoparticle size, composition and structure. The size of the bimetallic particles is determined by the total number of ALD cycles performed. The composition is dictated by the relative number of ALD cycles used for each component. Finally, the structure of the bimetallic nanoparticles is controlled by the order in which the individual cycles are executed. In situ FTIR measurements of CO chemisorption for the first time directly demonstrated this capability by mapping the atomic-scale evolution in the surface composition during bimetallic nanoparticle synthesis. During the growth of a Pt shell on a Pd/Al 2 O 3 catalyst, the gradual decrease of bridge-bonded CO on Pd (1,917 cm −1 ) and simultaneous increase of the linear CO on Pt provide direct evidence for the reduction in surface Pd concentration with increasing Pt ALD cycles ( Fig. 3a ). The completion of a continuous Pt shell on the Pd nanoparticle core occurred after ~10 Pt ALD cycles (~1.5 ML), as indicated by the disappearance of the bridge-bonded CO peak on Pd. Consequently, the Pt shell thickness on Pd nanoparticles can be precisely tuned by ~0.15 ML per cycle. Figure 3 demonstrates that the structure of the PdPt bimetallic nanoparticles can be controlled to be either core-shell or well-mixed alloy by tailoring the Pd and Pt ALD sequence, and this is corroborated by the HAADF-STEM measurements ( Fig. 4 ). It is noteworthy that these synthesized ALD bimetallic nanoparticles are rather structurally and thermally stable at temperatures below 300 °C in both oxidizing and reducing environments, which is very important for practical catalytic applications. In conclusion, low temperature selective metal ALD is a versatile and powerful method for synthesizing supported, bimetallic nanoparticles. The self-limiting feature of ALD, combined with careful selection of the metal ALD co-reactants and deposition temperature, and the implementation of tailored ALD pulse sequences allow atomically precise control over the nanoparticle size, composition and structure. Having demonstrated this capability for all combinations of three metals on three metal oxide supports, it is likely that these methods are general and will apply to a broad range of other ALD metals and supports ( Supplementary Fig. 14 ). In situ CO chemisorption FTIR is shown to be a powerful characterization tool to infer nanoparticle structure and composition as verified by STEM analysis. Although the economics of this methodology would need to be carefully considered before commercial application, ALD could complement other catalyst synthesis methods and offers a promising alternative synthetic route to supported bimetallic or multi-metallic catalysts. Metal ALD ALD was performed in a custom viscous flow stainless tube reactor system, using ultrahigh purity N 2 (UHP, 99.999%) carrier gas at a flow rate of 300 sccm and a pressure of 1 Torr [48] . Pd ALD utilized Pd(hfac) 2 (Sigma-Aldrich, >97%) and either formalin (Sigma-Aldrich) or H 2 (refs 28 , 45 ). The Pd(hfac) 2 was contained in a stainless steel bubbler heated to 60 °C. Pt ALD was conducted using MeCpPtMe 3 (Sigma-Aldrich, 98%) heated to 50 °C and either O 3 or O 2 . Ru ALD was conducted via an ABC process using Ru(EtCp) 2 (Sigma-Aldrich, 98%) heated to 80 °C, 99.999% O 2 and 99.99% H 2 at 150 or 200 °C. The ALD timing sequences are expressed as t 1 –t 2 –t 3 –t 4 , corresponding to the metal precursor exposure time, the metal precursor purge time, the coreactant exposure time and the coreactant purge time, respectively, with all times in seconds (s). Similarly the ABC-type ALD timing sequences are expressed as t 1 –t 2 –t 3 –t 4 –t 5 –t 6 . In situ QCM measurements We employed in situ QCM to investigate the metal ALD on both metal and oxide surfaces [26] , [48] , [49] . To examine the metal ALD on the Al 2 O 3 , TiO 2 and ZrO 2 surfaces, ~10 nm of the oxide film was deposited on the QCM sensor by ALD before the metal ALD. The Al 2 O 3 ALD used trimethylaluminum (TMA, Sigma-Aldrich, 97%) and water ( 1-5-1-5 ); the TiO 2 ALD used titanium tetraisopropoxide (TTIP, Sigma-Aldrich, 97%) and water ( 2-5-2-5 ); and the ZrO 2 ALD used tetrakis(dimethylamido)zirconium(IV) (TDMAZr, Sigma-Aldrich) and water ( 3-5-3-5 ). The TMA reservoir was held at room temperature, while the TTIP and TDMAZr bubblers were both heated to 80 °C. To examine metal ALD on the Ru, Pt and Pd surfaces, ~5–10 nm of the primary metal was first deposited on the QCM sensor by ALD, after which the secondary metal ALD was performed. The timing sequences were ( 5-5-5-5 ) for the Pd ALD (Pd(hfac) 2 +HCHO (or H 2 )), ( 2-5-5-5 ) for the Pt ALD (MeCpPtMe 3 +O 2 ) and ( 3-5-5-10-5-5 ) for the Ru ALD (Ru(EtCp) 2 +O 2 +H 2 ). In situ CO chemisorption FTIR In situ CO chemisorption FTIR measurements were conducted to investigate the evolution of the surface composition after every ALD cycle of the secondary metal on the primary metal nanoparticles. The custom ALD-FTIR chamber consisted of a stainless steel cross with a pair of IR-transmissive KBr windows installed on opposite flanges with gate valves to protect the windows from the ALD coatings. The sample pellet was positioned in the center of the cross in the path of the IR beam and was prepared by pressing the spherical alumina powder (NanoDur, 99.5%, Alfa Aesar) into a stainless steel grid (Fotofab, Chicago, IL). The FT-IR spectra were recorded using a Thermo Scientific Nicolet 6700 FT-IR spectrometer with an MCT detector. A typical FTIR spectrum was recorded at 4 cm −1 resolution using 256 scans. The FTIR chamber was heated to 150 °C to minimize condensation during the ALD and maintained at 1 Torr pressure with a flow of 300 sccm UHP N 2 . The ALD nanoparticle sample was first calcined in ~10% O 2 flow at 200 °C for 30 min then reduced in ~10% H 2 at 150 °C for another 30 min. An IR background spectrum was then collected under pure N 2 flow. After closing the two IR-window gate valves, CO (Matheson, research purity, 99.998%) was dosed for 60 s at a partial pressure of 0.3 Torr to saturate the ALD metal nanoparticle sample. Next, the ALD chamber was purged for 30 s to remove the gas phase CO. The two IR-window gate valves were then opened, and an IR spectrum was collected for the starting metal nanoparticles. To remove the chemisorbed CO and regenerate the clean metal surface, O 2 was dosed for 120 s at a partial pressure of 0.2 Torr, followed by a 30 s N 2 purge, and then H 2 was dosed for 120 s at a partial pressure of 0.2 Torr. Next, ALD of the secondary metal was performed for a certain number of ALD cycles, and the procedure of CO chemisorption, FTIR, O 2 burning and H 2 reduction was repeated. In the case of Pt shell growth on the Pd nanoparticles, the H 2 reduction step after CO burning was skipped since surface oxygen serves as the active site in Pt ALD. The timing sequences for the Pd, Pt and Ru ALD were ( 80-60-120-60 ), ( 70-60-120-30 ) and ( 120-60-60-60-60-60 ), respectively. In situ CO chemisorption FTIR measurements were also used to investigate the thermal stability of ALD bimetallic nanoparticles. For the well-mixed 12Pt10Pd alloy sample, the thermal treatment was first carried out in N 2 at 150 °C for 14 h, then in either 10% O 2 or 10% H 2 at 250, 300 and 400 °C for 1 h. The CO chemisorption spectra were collected at 150 °C after each treatment step. In the case of 1Pt-core 35Ru-rich-shell sample, it was treated in either 10% O 2 or 10% H 2 at 250, 300 and 350 °C for 1 h, and then the CO chemisorption spectra were collected at 200 °C after each treatment step. STEM HAADF-STEM imaging was performed using a JEOL JEM-ARM200CF probe aberration-corrected cold-field emission STEM operating at 200 kV with a point-resolution of less than 0.08 nm. X-ray energy-dispersive spectroscopy (XEDS) experiments were performed using the same STEM instrument that is equipped with an Oxford Instrument’s X-Max 80 mm 2 silicon-drift detector. The line profile analysis was performed on multiple particles for each sample. The STEM instrument is located in the Research Resources Center at University of Illinois at Chicago. How to cite this article: Lu, J. et al. Toward atomically-precise synthesis of supported bimetallic nanoparticles using atomic layer deposition. Nat. Commun. 5:3264 doi: 10.1038/ncomms4264 (2014).